Zic1 controls placode progenitor formation non-cell autonomously by regulating retinoic acid production and transport All cranial placode progenitors arise from a common precursor field anterior to the neural plate, the pre-placodal region (PPR). We showed that transcription factor Zic1, expressed at the anterior neural plate, is necessary and sufficient to promote placode fate. Here we reveal the non-cell autonomous activity of Zic1 and implicate retinoic acid (RA) signalling as a key player in cranial placode progenitor specification. In a screen for genes activated by Zic1, we identify several factors involved in RA metabolism and function. Among them we show that retinaldehyde dehydrogenase 2 (RALDH2) and lipocalin-type prostaglandin D2 synthase (LPGDS), which, respectively, regulate the synthesis and transport of RA, directly participate in the establishment of the PPR. We propose that RALDH2 and LPGDS induction by Zic1 at the anterior neural plate allows for the localized production and transport of RA, which in turn activates a cranial placode developmental programme in neighbouring cells. Cranial sensory placodes are thickenings of the embryonic head ectoderm that give rise to the specialized paired sense organs and sensory cranial ganglia. While they produce very diverse cell types such as sensory neurons, lens fibres and hormone-secreting cells [1] , [2] , [3] , all placode progenitors arise from a common precursor field that borders the anterior neural plate known as the pre-placodal region (PPR). Subsequently, in response to inductive interactions with surrounding tissues the PPR divides into territories with distinct identities to generate the adenohypophyseal, olfactory, lens, trigeminal, otic and epibranchial placodes. Placode progenitors are induced by a combination of inductive signals primarily mediated by fibroblast growth factor (FGF) and attenuation of bone morphogenetic protein (BMP) and Wnt signals [4] , [5] , [6] . The zinc-finger transcription factor, Zic1, is one of the earliest genes activated in response to these signalling events, and in Xenopus , Zic1 is both necessary and sufficient to promote placodal fate by regulating the expression of the PPR-specific genes, Six1 and Eya1 (ref. 7 ). Interestingly, Zic1 is expressed at the anterior neural plate but does not overlap with the prospective PPR [8] , [9] , suggesting that Zic1 regulates placode formation in a non-cell autonomous manner. To gain insights into the mechanisms by which Zic1 regulates PPR formation, we performed a microarray analysis to identify genes activated by Zic1 in a Xenopus animal explant assay. Among the targets regulated by Zic1, we found a number of genes involved in the synthesis and metabolism of retinoic acid (RA) including lipocalin-type prostaglandin D2 synthase ( LPGDS ), retinaldehyde dehydrogenase 2 ( RALDH2 ), two members of the cytochrome P450 enzyme family ( Cyp26a and Cyp26c ) and a cellular RA-binding protein 2 ( Crabp2 ) signifying the importance of this signalling pathway in placode formation. Here we present evidence that Zic1 regulates placode progenitor formation non-cell autonomously by controlling RA production and transport at the anterior neural plate. Identification of downstream targets of Zic1 The transcription factor Zic1 is expressed at the anterior neural plate [7] , [8] , [9] , [10] and is required for the formation of sensory placode progenitors [7] . To gain insights into the mechanisms by which Zic1 regulates sensory placode formation, we performed a microarray screen to identify targets of Zic1 (ref. 11 ). The screen was based on the observation that while expression of Zic1 favoured placode fate in Xenopus animal cap explants, simultaneous expression of Pax3 repressed placode-specific genes to promote neural crest fate [7] , [11] ( Fig. 1a ). Among the genes that were both strongly upregulated by Zic1, as compared with Pax3 alone, and repressed by Pax3 co-injection, we found several well-characterized early placode-specific genes, including Six1 , Eya1 , Xanf1 , Ebf2 and Sox11 ( Fig. 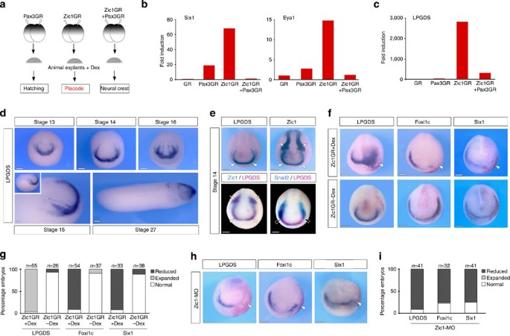Figure 1: LPGDS is a downstream target of Zic1. (a) Experimental design for the selection of Zic1 targets. (b) Fold induction ofSix1,Eya1and (c)LPGDSfrom the microarray data. (d)In situhybridization forLPGDS(stages 13, 14 and 16 are frontal views; stage 15 and stage 27 are lateral views, anterior to right, dorsal to top). (e)In situhybridization forLPGDSandZic1in stage-matched embryos (upper panels).LPGDSandZic1co-localize at the anterior neural plate (arrowheads), while Zic1 is also expressed in neural crest progenitors (arrows). Doublein situhybridization (lower panels) shows overlapping expression ofLPGDSandZic1at the anterior neural plate (arrowheads; left panel), whileLPGDSandSnail2(right panel) have adjacent but non-overlapping expression domains (black arrowheads). Frontal views. (f) In embryos injected with Zic1GR mRNA and treated with dexamethasone (+Dex),LPGDSis markedly expanded (arrowhead), whileFoxi1candSix1expression at the PPR are reduced (arrowheads). The same injection in the absence of dexamethasone (−Dex) had no effect on the expression of these genes. Frontal views, the injected side is indicated by the lineage tracer (Red-Gal). (g) Quantification of the Zic1GR injection results. Three independent experiments were performed. The number of embryos analysed (n) is indicated on the top of each bar. (h) Zic1 knockdown (Zic1-MO injection) reducesLPGDS,Foxi1candSix1expression. (i) Quantification of the Zic1-MO injection results. Three independent experiments were performed. The number of embryos analysed (n) is indicated on the top of each bar. Scale bars, 200 μm. 1b ; Supplementary Table 1 ). The recovery of these genes was an important validation of our experimental design. We also found several novel potential regulators of placode formation ( Supplementary Table 1 ). These genes were initially screened by whole-mount in situ hybridization to select factors expressed at the anterior neural plate, in a pattern similar to Zic1 . One candidate that fulfilled this criterion was LPGDS ( Fig. 1c ), also known as Cpl1 (refs 12 , 13 , 14 , 15 ). By in situ hybridization LPGDS is first expressed at stage 13 in the anterior region of the neural plate ( Fig. 1d ). This expression pattern is maintained throughout neurulation and then appears confined to the head region in tailbud stage embryos ( Fig. 1d ). Double in situ hybridization demonstrates that LPGDS completely overlaps with the anterior expression domain of Zic1 ( Fig. 1e ), but is excluded from the lateral expression domain of Zic1, which corresponds to the prospective neural crest region. In situ hybridization for the neural crest-specific gene Snail2 (ref. 16 ) confirmed that there is no overlap between LPGDS expression domain and neural crest progenitors; LPGDS abuts the anterior expression domain of Snail2 ( Fig. 1e ). Figure 1: LPGDS is a downstream target of Zic1. ( a ) Experimental design for the selection of Zic1 targets. ( b ) Fold induction of Six1 , Eya1 and ( c ) LPGDS from the microarray data. ( d ) In situ hybridization for LPGDS (stages 13, 14 and 16 are frontal views; stage 15 and stage 27 are lateral views, anterior to right, dorsal to top). ( e ) In situ hybridization for LPGDS and Zic1 in stage-matched embryos (upper panels). LPGDS and Zic1 co-localize at the anterior neural plate (arrowheads), while Zic1 is also expressed in neural crest progenitors (arrows). Double in situ hybridization (lower panels) shows overlapping expression of LPGDS and Zic1 at the anterior neural plate (arrowheads; left panel), while LPGDS and Snail2 (right panel) have adjacent but non-overlapping expression domains (black arrowheads). Frontal views. ( f ) In embryos injected with Zic1GR mRNA and treated with dexamethasone (+Dex), LPGDS is markedly expanded (arrowhead), while Foxi1c and Six1 expression at the PPR are reduced (arrowheads). The same injection in the absence of dexamethasone (−Dex) had no effect on the expression of these genes. Frontal views, the injected side is indicated by the lineage tracer (Red-Gal). ( g ) Quantification of the Zic1GR injection results. Three independent experiments were performed. The number of embryos analysed ( n ) is indicated on the top of each bar. ( h ) Zic1 knockdown (Zic1-MO injection) reduces LPGDS , Foxi1c and Six1 expression. ( i ) Quantification of the Zic1-MO injection results. Three independent experiments were performed. The number of embryos analysed ( n ) is indicated on the top of each bar. Scale bars, 200 μm. Full size image To further establish that LPGDS is a true target of Zic1, we analysed LPGDS expression pattern in embryos injected with Zic1GR messenger RNA (mRNA) (a hormone-inducible version of Zic1 fused to human glucocorticoid receptor (GR) ligand-binding domain), or a morpholino antisense oligonucleotide that blocks Zic1 function (Zic1-MO) [7] , [9] . In embryos injected with Zic1GR mRNA and treated with dexamethasone, we observed a marked upregulation and expansion of the LPGDS expression domain ( Fig. 1f,g ). The same injection in the absence of dexamethasone had no effect on LPGDS expression ( Fig. 1f,g ). Conversely, injection of Zic1-MO completely inhibited LPGDS expression on the injected side ( Fig. 1h,i ). Interestingly, in both situations we observed a reduction of Foxi1c and Six1 expression, two early PPR-specific genes ( Fig. 1f–i ). These observations confirm that LPGDS is a downstream target of Zic1 and indicate that placode formation is sensitive to Zic1 and LPGDS expression levels in the embryos. LPGDS is required for placode formation The expression pattern of LPGDS at the anterior neural plate and its regulation by Zic1 suggest a potential role in placode formation. To test this possibility, we used a translation-blocking morpholino antisense oligonucleotide (LPGDS-MO) to interfere with LPGDS function. The activity of the morpholino was confirmed in an in vitro transcription/translation assay in which LPGDS-MO blocked LPGDS protein production ( Fig. 2a ; Supplementary Fig. 1 ). Unilateral injection of LPGDS-MO (40 ng) in the animal pole region of two-cell stage embryos resulted in a marked decrease expression of Six1 (refs 17 , 18 ), Foxi1c [18] , [19] and Sox2 (ref. 20 ), three genes broadly expressed at the PPR ( Fig. 2b,d ). We also analysed the expression of genes restricted to individual placodal domains such as Dmrt4 for the adenohypophyseal and olfactory placodes [21] , Pax8 for the otic and lateral line placodes [22] and Tbx2 for otic and trigeminal/profundal placodes [23] . For each one of these genes a significant reduction of expression was observed on the injected side ( Fig. 2c ) in >80% of the embryos ( Fig. 2d ). Injection of a control morpholino (Cont-MO) had no effect on the expression of these genes ( Supplementary Fig. 2e ). To further establish the specificity of LPGDS knockdown phenotype, we used a second morpholino (LPGDS-MO2) that specifically interfered with LPGDS pre-mRNA splicing by targeting intron 1/exon 2 junction ( Supplementary Fig. 2a ), resulting in the production of a transcript of higher size, due to intron retention ( Supplementary Fig. 2b ). The phenotype of LPGDS-MO2-injected embryos was indistinguishable from the phenotype generated by injection of the translation-blocking morpholino, with inhibition of Foxi1c , Six1 and Dmrt4 , although at a lower frequency ( Supplementary Fig. 2c,d ). These results indicate that LPGDS is critically required for the establishment of the PPR and for sensory placode formation. 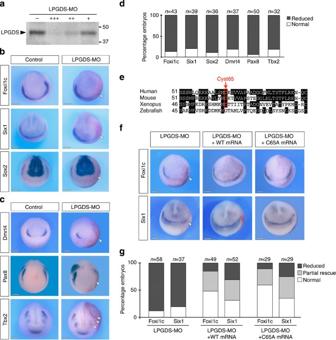Figure 2: LPGDS is required for placode development. (a) Increasing amounts of LPGDS-MO 10 ng (+), 100 ng (++) and 1,000 ng (+++) blocks translation directed byLPGDSmRNA in anin vitrocoupled transcription/translation reaction. The position of markers of known molecular weight (kDa) is indicated. (b)In situhybridization for pan-placodal and (c) placode-specific genes in control and LPGDS-MO-injected embryos (frontal views, dorsal to top). Arrowheads indicate reduced expression on the injected side. (d) Quantification of the results. Four independent experiments were performed. The number of embryos analysed (n) is indicated on the top of each bar. (e) Amino-acid sequence alignment showing the conserved cysteine residue (Cyst65), centre of LPGDS enzymatic activity. (f)Foxi1candSix1expression domains are rescued in LPGDS-MO-injected embryos by co-injection of either WT or C65A mouseLPGDSmRNA. Frontal views, dorsal to top; injected side is indicated by the lineage tracer (Red-Gal). (g) Quantification of the rescue experiment. Three independent experiments were performed. The number of embryos analysed (n) is indicated on the top of each bar. LPGDS-MO vs LPGDS-MO+WT or LPGDS-MO+C65A mRNA-injected embryos (P<0.001, Fisher’s exact test.); LPGDS-MO+WT mRNA vs LPGDS-MO+C65A mRNA-injected embryos show no significant differences. Scale bars, 200 μm. Figure 2: LPGDS is required for placode development. ( a ) Increasing amounts of LPGDS-MO 10 ng (+), 100 ng (++) and 1,000 ng (+++) blocks translation directed by LPGDS mRNA in an in vitro coupled transcription/translation reaction. The position of markers of known molecular weight (kDa) is indicated. ( b ) In situ hybridization for pan-placodal and ( c ) placode-specific genes in control and LPGDS-MO-injected embryos (frontal views, dorsal to top). Arrowheads indicate reduced expression on the injected side. ( d ) Quantification of the results. Four independent experiments were performed. The number of embryos analysed ( n ) is indicated on the top of each bar. ( e ) Amino-acid sequence alignment showing the conserved cysteine residue (Cyst65), centre of LPGDS enzymatic activity. ( f ) Foxi1c and Six1 expression domains are rescued in LPGDS-MO-injected embryos by co-injection of either WT or C65A mouse LPGDS mRNA. Frontal views, dorsal to top; injected side is indicated by the lineage tracer (Red-Gal). ( g ) Quantification of the rescue experiment. Three independent experiments were performed. The number of embryos analysed ( n ) is indicated on the top of each bar. LPGDS-MO vs LPGDS-MO+WT or LPGDS-MO+C65A mRNA-injected embryos ( P <0.001, Fisher’s exact test. ); LPGDS-MO+WT mRNA vs LPGDS-MO+C65A mRNA-injected embryos show no significant differences. Scale bars, 200 μm. Full size image LPGDS functions independently of its enzymatic activity LPGDS has a dual function, as an enzyme involved in the biosynthesis of prostaglandin D2 (PGD2) from its precursor, and as a lipophilic ligand-binding protein when secreted [24] . The LPGDS molecule contains three cysteine residues, and site-directed mutagenesis has established that the cysteine residue at position 65 (Cyst65) is essential for the enzymatic activity of LPGDS [25] , a cysteine highly conserved from human to frogs ( Fig. 2e ). To determine whether LPGDS regulates placode formation through PGD2 signalling, we performed a rescue experiment using mRNA encoding wild-type (WT) mouse LPGDS or a mutated version in which Cyst65 has been replaced by an alanine (C65A), thereby completely abolishing the enzymatic activity of LPGDS [25] . Embryos at the two-cell stage were sequentially injected with LPGDS-MO and either with WT or C65A mouse LPGDS mRNA. Both mRNA were equally efficient at rescuing Foxi1c and Six1 expression in morphant embryos ( Fig. 2f,g ). Complementary to this rescue assay, we found that well-characterized pharmacological agents that specifically block the PGD2 signalling pathway did not affect Foxi1c expression at the PPR ( Supplementary Fig. 3 ). Altogether, these results demonstrate that LPGDS regulates placode formation through a mechanism that does not involve its enzymatic activity and the production of PGD2. LPGDS functions as a carrier for RA Since LPGDS binds retinoids with high affinity [14] , [26] , we wished to determine whether LPGDS regulated placode formation through this mechanism. As a preliminary evaluation, we treated intact embryos at the gastrula stage (stage 11) with increasing doses of RA (0.01–10 μM) and analysed the consequence on PPR formation. We found that the lower doses of RA (0.01 and 0.1 μM) resulted in an expansion of Foxi1c and Six1 expression domains, while the higher doses of RA (1 and 10 μM) inhibited the expression of both genes ( Fig. 3 ), indicating that PPR formation is very sensitive to RA levels in the embryo. On the basis of these observations, we performed a rescue experiment in which LPGDS-MO-injected embryos were exposed at stage 11 to 0.1 μM of RA (the dose of RA that promotes strong expansion of PPR genes; Fig. 3 ) or a RA receptor (RAR) agonist, TTNPB [27] . Both treatments efficiently rescued Foxi1c and Six1 expression in morphant embryos and occasionally expanded Foxi1c and Six1 expression on the control side ( Fig. 4a,b ). LPGDS can also bind retinaldehyde (retinal), the RA precursor, with high affinity [14] , [26] ; however, this compound was unable to rescue the Foxi1c expression domain in LPGDS-depleted embryos ( Supplementary Fig. 4 ), indicating that in the context of PPR formation LPGDS is functioning primarily as a RA carrier, and that RA is the active compound promoting PPR formation. 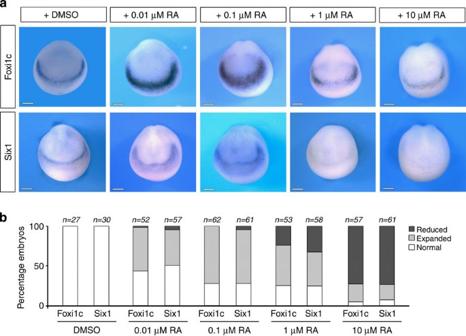Figure 3: Retinoic acid affects PPR formation in a dose-dependent manner. (a) Treatment of intact embryos at stage 11 with increasing doses of RA (0.01, 0.1, 1 and 10 μM) disruptsFox1icandSix1expression at the PPR. Dimethylsulphoxide (DMSO) was used as a control. Frontal views, dorsal to top. (b) Quantification of the results. Four independent experiments were performed. The number of embryos analysed for each condition (n) is indicated on the top of each bar. Scale bars, 200 μm. Figure 3: Retinoic acid affects PPR formation in a dose-dependent manner. ( a ) Treatment of intact embryos at stage 11 with increasing doses of RA (0.01, 0.1, 1 and 10 μM) disrupts Fox1ic and Six1 expression at the PPR. Dimethylsulphoxide (DMSO) was used as a control. Frontal views, dorsal to top. ( b ) Quantification of the results. Four independent experiments were performed. The number of embryos analysed for each condition ( n ) is indicated on the top of each bar. Scale bars, 200 μm. 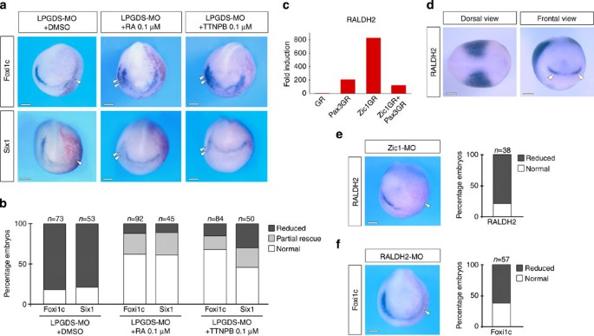Figure 4: Retinoic acid signalling regulates placode formation. (a) Treatment at stage 11 of LPGDS-depleted embryos (LPGDS-MO) with 0.1 μM RA or with the RA receptor agonist, TTNPB, restored completely or partiallyFoxi1candSix1expression on the injected side. Frontal views, dorsal to top. Injected side is indicated by the lineage tracer (Red-Gal). Double arrowheads indicateFoxi1corSix1expansion on the control side. (b) Quantification of the rescue experiment. Four independent experiments were performed. The number of embryos analysed for each condition (n) is indicated on the top of each bar. Dimethylsulphoxide (DMSO) vs RA- or TTNPB-treated embryos (P<0.001, Fisher’s exact test) RA- vs TTNPB-treated embryos show no significant differences. (c) Fold induction ofRALDH2from the microarray data. (d) Byin situhybridizationRALDH2is detected in the trunk mesoderm (dorsal view, anterior to right) and at the anterior neural plate (frontal view; arrowheads). (e)RALDH2expression is lost in Zic1-depleted embryos. The graph is a quantification of the results. Three independent experiments were performed. The number of embryos analysed (n) is indicated on the top of the bar. (f)Foxi1cexpression is reduced in RALDH2-MO-injected embryos. The graph is a quantification of the results. Three independent experiments were performed. The number of embryos analysed (n) is indicated on the top of the bar. (e,f) Arrowheads indicate reduced expression on the injected side. Scale bars, 200 μm. Full size image Figure 4: Retinoic acid signalling regulates placode formation. ( a ) Treatment at stage 11 of LPGDS-depleted embryos (LPGDS-MO) with 0.1 μM RA or with the RA receptor agonist, TTNPB, restored completely or partially Foxi1c and Six1 expression on the injected side. Frontal views, dorsal to top. Injected side is indicated by the lineage tracer (Red-Gal). Double arrowheads indicate Foxi1c or Six1 expansion on the control side. ( b ) Quantification of the rescue experiment. Four independent experiments were performed. The number of embryos analysed for each condition ( n ) is indicated on the top of each bar. Dimethylsulphoxide (DMSO) vs RA- or TTNPB-treated embryos ( P <0.001, Fisher’s exact test) RA- vs TTNPB-treated embryos show no significant differences. ( c ) Fold induction of RALDH2 from the microarray data. ( d ) By in situ hybridization RALDH2 is detected in the trunk mesoderm (dorsal view, anterior to right) and at the anterior neural plate (frontal view; arrowheads). ( e ) RALDH2 expression is lost in Zic1-depleted embryos. The graph is a quantification of the results. Three independent experiments were performed. The number of embryos analysed ( n ) is indicated on the top of the bar. ( f ) Foxi1c expression is reduced in RALDH2-MO-injected embryos. The graph is a quantification of the results. Three independent experiments were performed. The number of embryos analysed ( n ) is indicated on the top of the bar. ( e , f ) Arrowheads indicate reduced expression on the injected side. Scale bars, 200 μm. Full size image Zic1 regulates RALDH2 expression Our results suggest that LPGDS activity at the anterior neural plate is linked to RA activity. Consistent with this observation, we found several components of RA metabolism and function strongly upregulated by Zic1 in the microarray screen ( Supplementary Table 1 ). These include RALDH2 , the enzyme responsible for the synthesis of RA from its precursor retinal, two RA-degrading enzymes ( Cyp26a and Cyp26c ) and a cellular RA-binding protein 2 ( Crabp2 ). In the microarray samples, RALDH2 induction levels followed the same pattern as LPDGS ( Fig. 4c ). RALDH2 is expressed in the trunk mesoderm, as well as in a discrete U-shaped ectodermal domain around the anterior neural plate, similar to LPGDS ( Fig. 4d ) [28] . Zic1 knockdown reduced RALDH2 expression in the embryo ( Fig. 4e ), confirming that RALDH2 is functioning downstream of Zic1. Moreover, in the absence of RALDH2 function, Foxi1c was severely reduced at the PPR ( Fig. 4f ), further demonstrating the link between Zic1, RALDH2 activity and placode formation. Zic1 induces placode fate non-cell autonomously Our data indicate that Zic1 may control RA signalling at the anterior neural plate through the activation of RALDH2 to produce RA and LPGDS to transport RA extracellularly. Zic1 , RALDH2 and LPGDS are all confined to the anterior neural plate, at a distance from the prospective PPR ( Foxi1c- expressing cells; Fig. 5a ), suggesting that Zic1 regulates placode formation non-cell autonomously. To test this possibility, embryos were injected in one blastomere at the two-cell stage with Zic1GR mRNA and mRNA encoding the lineage tracer green fluorescent protein (GFP), animal explants isolated at the blastula stage, treated with dexamethasone and cultured for 8 h ( Fig. 5b ). Injection of GR mRNA was used as a negative control ( Supplementary Fig. 5 ). Explants were then processed for in situ hybridization on sections. In these explants, Six1 and Foxi1c expression was exclusively confined to GFP-negative cells, derived from the uninjected blastomere ( Fig. 5c ; upper panels). By contrast, LPGDS and RALDH2 expression was always closely associated with Zic1GR/GFP-positive cells ( Fig. 5c ; lower panels). Altogether, these results demonstrate that Zic1 is inducing placode fate by a non-cell autonomous mechanism involving activation of RA signalling. 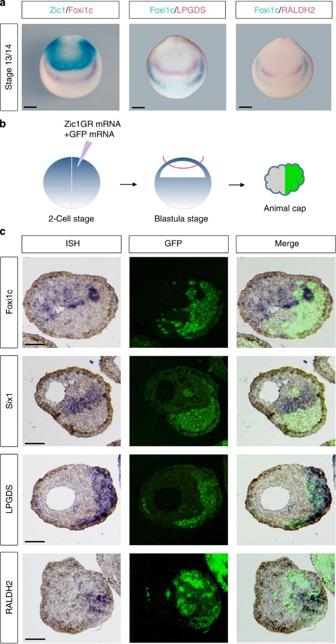Figure 5: Zic1 regulates placode formation non-cell autonomously. (a) Doublein situhybridization forZic1/Foxi1c,Foxi1c/LPGDSandFoxi1c/RALDH2showing thatZic1,LPGDSandRALDH2are expressed at a distance from the PPR (Foxi1c-expressing cells). Frontal views, dorsal to top. Scale bars, 200 μm. (b) Animal explants dissected from embryos injected in one blastomere at the two-cell stage with Zic1GR and GFP mRNAs were cultured for 8 h in dexamethasone and analysed byin situhybridization (ISH). (c) ISH forFoxi1c,Six1,LPGDSandRALDH2on sections of animal explants derived from embryos injected withZic1GRandGFPmRNA in one blastomere at the two-cell stage (left panels). In each case the Zic1GR-expressing cells (GFP positive) are shown (middle panels). Merge of fluorescence and ISH images (right panels). Three independent experiments were performed with similar results for each probe as pictured (Foxi1c,n=14;Six1,n=13;LPGDS,n=13 andRALDH2,n=11). Scale bars, 100 μm. Figure 5: Zic1 regulates placode formation non-cell autonomously. ( a ) Double in situ hybridization for Zic1/Foxi1c , Foxi1c/LPGDS and Foxi1c/RALDH2 showing that Zic1 , LPGDS and RALDH2 are expressed at a distance from the PPR ( Foxi1c- expressing cells). Frontal views, dorsal to top. Scale bars, 200 μm. ( b ) Animal explants dissected from embryos injected in one blastomere at the two-cell stage with Zic1GR and GFP mRNAs were cultured for 8 h in dexamethasone and analysed by in situ hybridization (ISH). ( c ) ISH for Foxi1c , Six1 , LPGDS and RALDH2 on sections of animal explants derived from embryos injected with Zic1GR and GFP mRNA in one blastomere at the two-cell stage (left panels). In each case the Zic1GR-expressing cells (GFP positive) are shown (middle panels). Merge of fluorescence and ISH images (right panels). Three independent experiments were performed with similar results for each probe as pictured ( Foxi1c , n =14; Six1 , n =13; LPGDS , n =13 and RALDH2 , n =11). Scale bars, 100 μm. Full size image Zic1-activated RA signalling uses non-canonical RARs To further establish that the placode-inducing activity of Zic1 depends on active RA signalling, we analysed by reverse transcription (RT)–PCR the expression of Six1 and Eya1 in Zic1GR-injected animal explants treated with 100 μM of disulfiram or citral ( Fig. 6a ), two general inhibitors of alcohol and aldehyde dehydrogenases [29] , [30] , the group of enzymes that sequentially catalyse the oxidation of retinol and retinaldehyde to produce RA. In these animal explants treated with the inhibitors, the induction of Six1 and Eya1 by Zic1GR was significantly reduced ( Fig. 6b ; Supplementary Fig. 6a,b ), consistent with the view that placode induction by Zic1 depends on RA production. 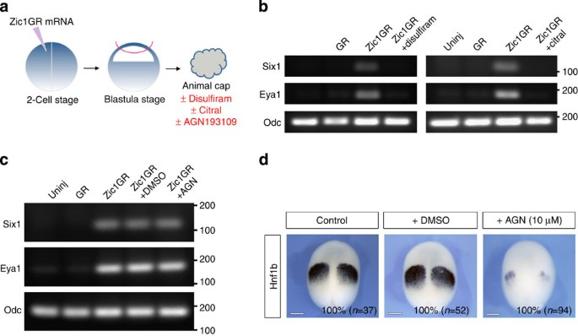Figure 6: Zic1 regulates placode fate independently of canonical RA receptors. (a) Animal explants dissected from embryos injected in one blastomere at the two-cell stage with Zic1GR mRNA and cultured for 8 h in dexamethasone, with or without the pharmacological inhibitors disulfiram (100 μM), citral (100 μM) or AGN193109 (10 μM). (b) RT–PCR analysis ofSix1andEya1expression in animal explants expressing Zic1GR treated with disulfiram or citral.Odc(ornithine decarboxylase) is shown as a loading control. Controls are uninjected (Uninj) and GR mRNA-injected (GR) animal explants. Similar results were obtained in four independent experiments for each inhibitor. The position of markers of known size is indicated (bp). (c) RT–PCR analysis ofSix1andEya1expression in Zic1GR-injected animal explants treated with the pan-RAR antagonist, AGN193109. Controls are uninjected (Uninj), GR mRNA-injected (GR) and Zic1GR mRNA-injected treated with dimethylsulphoxide (+DMSO) animal explants. Similar results were obtained in six independent experiments. The position of markers of known size is indicated (bp). (d) AGN193109 treatment blocksHnf1bexpression in the posterior hindbrain (100% of the embryos;n=94), while in DMSO-treated embryosHnf1bexpression is similar to that of control embryos (100% of the embryos;n=52 andn=37, respectively). Three independent experiments were performed. Stage 13 embryos, dorsal views, anterior to top. Scale bars, 200 μm. Figure 6: Zic1 regulates placode fate independently of canonical RA receptors. ( a ) Animal explants dissected from embryos injected in one blastomere at the two-cell stage with Zic1GR mRNA and cultured for 8 h in dexamethasone, with or without the pharmacological inhibitors disulfiram (100 μM), citral (100 μM) or AGN193109 (10 μM). ( b ) RT–PCR analysis of Six1 and Eya1 expression in animal explants expressing Zic1GR treated with disulfiram or citral. Odc (ornithine decarboxylase) is shown as a loading control. Controls are uninjected (Uninj) and GR mRNA-injected (GR) animal explants. Similar results were obtained in four independent experiments for each inhibitor. The position of markers of known size is indicated (bp). ( c ) RT–PCR analysis of Six1 and Eya1 expression in Zic1GR-injected animal explants treated with the pan-RAR antagonist, AGN193109. Controls are uninjected (Uninj), GR mRNA-injected (GR) and Zic1GR mRNA-injected treated with dimethylsulphoxide (+DMSO) animal explants. Similar results were obtained in six independent experiments. The position of markers of known size is indicated (bp). ( d ) AGN193109 treatment blocks Hnf1b expression in the posterior hindbrain (100% of the embryos; n =94), while in DMSO-treated embryos Hnf1b expression is similar to that of control embryos (100% of the embryos; n =52 and n =37, respectively). Three independent experiments were performed. Stage 13 embryos, dorsal views, anterior to top. Scale bars, 200 μm. Full size image To determine whether the placode-inducing activity of Zic1 is mediated through canonical RARs, Zic1GR-injected animal explants were treated with a well-characterized pan-RAR antagonist, AGN193109 (refs 31 , 32 ) ( Fig. 6a ). Surprisingly, we found that AGN193109 was unable to block the expression of Six1 and Eya1 ( Fig. 6c ; Supplementary Fig. 6c ), while the same concentration of antagonist (10 μM) was extremely efficient at repressing Hnf1b expression in the whole embryo ( Fig. 6d ), a gene directly regulated by RAR signalling [33] . These results suggest that Zic1-activated RA signalling mediates its activity through a mechanism that does not involve canonical RARs, and may signal through other nuclear receptors that also bind RA, such as peroxisome proliferator-activated receptor β (ref. 34 ), and members of the RAR-related orphan receptors [35] , [36] . Our findings uncover the non-cell autonomous activity of Zic1 in the control of placode fate, and implicate RA signalling as a major player in cranial placode progenitor formation. We have identified several genes activated by Zic1 that are involved in RA metabolism and function. Among them we demonstrate that RALDH2 and LPGDS , respectively, are responsible for the synthesis and the transport of RA, and directly participate in the establishment of the PPR. We propose that the activation of RALDH2 and LPGDS at the anterior neural plate by Zic1 allows for the localized production and transport of RA, which in turn activates a placode developmental programme in neighbouring cells ( Fig. 7 ). 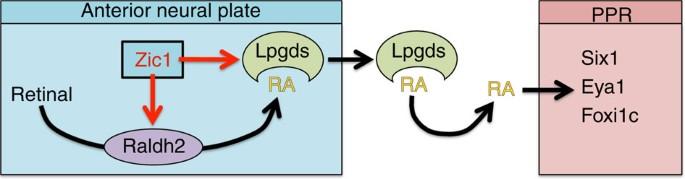Figure 7: Model for the regulation of PPR formation by Zic1 and RA signalling. Zic1 controls RA signalling at the anterior neural plate through the activation of RALDH2 to produce RA, and LPGDS to transport RA extracellularly. As a consequence, RA induces the expression ofSix1,Eya1andFoxi1cin neighbouring cells (PPR). Figure 7: Model for the regulation of PPR formation by Zic1 and RA signalling. Zic1 controls RA signalling at the anterior neural plate through the activation of RALDH2 to produce RA, and LPGDS to transport RA extracellularly. As a consequence, RA induces the expression of Six1 , Eya1 and Foxi1c in neighbouring cells (PPR). Full size image Xenopus LPGDS , also known as cpl1 (choroid plexus lipocalin 1), was first isolated in a screen for genes activated at gastrulation and specifically expressed in the nervous system [15] , and has been primarily used as a forebrain marker [12] , [13] , [37] . Its specific role at the anterior neural plate has not been studied. Cpl1/LPGDS was also isolated in another screen designed to identify direct targets of Zic1 (ref. 38 ); however, further studies are needed to confirm that Zic1 directly activates LPGDS expression. LPGDS is a bifunctional protein that acts as a PGD2-producing enzyme and a lipophilic ligand-binding protein [39] . More specifically, LPGDS can bind retinaldehyde and RA with high affinities [13] , [14] , [26] . In a rescue assay, using WT and mutant versions of mouse LPGDS we completely ruled out the involvement of its enzymatic activity, and demonstrated that LPGDS functions during placode formation through a mechanism implicating RA signalling. By exposing the entire embryo to RA, the expression of PPR genes was efficiently rescued in LPGDS-depleted embryos ( Fig. 4a,b ). In these experiments, the exogenous source of RA bypasses the requirement for an LPGDS-mediated transport of RA to the PPR. We posit that LPGDS is essential to transport RA outside the producing cells. LPGDS knockdown in the embryo leads to a loss of genes expressed at the PPR, as well as genes that are more specific for individual cranial placodes, suggesting a broad requirement for LPGDS and RA signalling in placode progenitor formation. A recent study has proposed that signalling through RARs (RARα2), which are expressed in the caudal half of the embryo [40] , was critical to set up the posterior boundary of the PPR [41] . Our experiments using the pan-RAR antagonist (AGN193109) suggest that the placode-inducing activity of Zic1 may use an RAR-independent pathway, pointing to the intriguing possibility that another set of receptors may mediate this activity. A similar activity of RA, independent of canonical RARs, has been described in the context of the developing mouse neural retina [42] . Several classes of nuclear receptors have been reported to bind RA, including peroxisome proliferator-activated receptor β (ref. 34 ) and members of the RAR-related orphan receptors [35] , [36] , and are therefore potential candidates to mediate the placode-inducing activity of Zic1. Future work will test this hypothesis. During embryonic development, RA signalling is essential for the regionalization of the embryo along the anteroposterior axis. Studies in several organisms have shown that RA is an important posteriorizing signal in all three germ layers, acting in concert with molecules of the Wnt and FGF families [43] , [44] , [45] . However, RA signalling may have a more direct role in PPR specification, independent of its posteriorizing activity, in a similar manner as the posteriorizing activity of FGF, and canonical Wnt can be uncoupled from their role in neural crest induction [10] , [46] . Consistent with this possibility, RALDH2 has two major expression domains in the early embryo: the paraxial and lateral plate mesoderm in the trunk region, as well as a discrete U-shaped ectodermal domain around the anterior neural plate [28] ( Fig. 4d ). While the former has been linked to the posteriorizing activity of RA, the later represents an independent source of RA, and we propose that this anterior domain is essential to pattern the cranial region of the embryo. In a recent study using novel transgenic RA sensor lines, RA activity has been visualized at the very anterior region of the zebrafish embryo and at the polster, and a candidate source of this activity is RALDH3 (ref. 47 ). In the mouse, RALDH2 is responsible for RA signalling in the early embryonic head, and knockout embryos die around E9.5–10.5 with severe forebrain and craniofacial defects [48] . In birds, RALDH3 is expressed anteriorly at early stages [49] , and vitamin A-deficient quail embryos have defective otic vesicles and lack the pituitary gland, two derivatives of cranial placodes [50] , [51] . Zic1 gain of function resulted in a marked upregulation of LPGDS in the embryo, which was surprisingly associated with a loss of early placode markers ( Six1 and Foxi1c ; Fig. 1f ). However, in light of our results linking Zic1 to RA signalling, this result is not completely unexpected and indicates that PPR formation is very sensitive to RA levels. As in other RA-regulated developmental processes, excess or insufficient RA signalling often result in similar outcomes [45] . Excess RA can shut down its own production through the downregulation of RALDH2 (ref. 52 ). Indeed, in embryos treated with RA, RALDH2 is preferentially lost anteriorly, leading to severe head truncation [28] . Furthermore, exposure of intact embryos to varying doses of RA affects PPR gene expression in a concentration-dependent manner ( Fig. 3 ). Altogether, these observations support the view that RA levels at the anterior neural plate are critical for placode formation. The non-cell autonomous activity of Zic1 in the control of placode fate was especially evident in the animal explant system ( Fig. 5 ). Interestingly, we never observed the activation of Six1 or Foxi1c in Zic1GR-expressing cells, rather the expression of Six1 and Foxi1c was always confined to adjacent cells, derived from the uninjected blastomere. A possible explanation is related to the activity of Cyp26c and Cyp26a, the RA-metabolizing enzymes, which were strongly upregulated by Zic1GR in the microarray. Typically, RA is released by RA-producing cells and can enter adjacent cells where it faces two scenarios: (i) in cells expressing Cyp26, RA is degraded preventing RA signalling and (ii) in cells that do not express Cyp26, RA enters the nucleus and initiates the transcription of target genes. It is possible that Cyp26 expression renders Zic1-expressing cells refractory to RA signalling, thereby allowing for the unidirectional propagation of the RA signal, and the establishment of sharp boundaries of gene expression. Consistent with this interpretation, in Xenopus Cyp26c is expressed in the neural plate but is excluded from the most anterior region of the embryo [53] . While the placode-inducing activity of Zic1 requires active RA signalling, RA is likely to act in concert with other signals to impart placode fate. Work in zebrafish suggests that Zic1 is functioning not only upstream of RA, but also by regulating Nodal and Hedgehog signalling to control midline tissue development in the head [54] , [55] . These factors are therefore good candidates to synergize with RA to promote cranial placode fate. Plasmids, constructs and oligonucleotides Xenopus laevis Pax3GR and Zic1GR , the hormone-inducible versions of Pax3 and Zic1, fused to the human glucocorticoid receptor (GR) ligand-binding domain [56] , wild type (WT) and mutated (C65A) mouse LPGDS (refs 7 , 25 ) were subcloned into pCS2+ expression plasmid. Pax3GR , Zic1GR , GR , WT and C65A mouse LPGDS , GFP and β -galactosidase mRNAs were synthesized in vitro using the Message Machine Kit (Ambion, Austin, TX). Zic1 (Zic1-MO) [9] , RALDH2 (RALDH2-MO) [29] and LPGDS (LPGDS-MO: 5′-TCAGAGCAAGCAAAATCCTCATCAT-3′; LPGDS-MO2: 5′-AGACCTAGAGGCAGAGAGAGGAATT-3′) morpholino antisense oligonucleotides were purchased from GeneTools (Philomath, OR). The specificity of the LPGDS-MO was tested in an in vitro transcription/translation-coupled rabbit reticulocyte lysate assay (Promega, Madison, WI). LPGDS-MO was designed to interfere with both LPGDS-a and LPGDS-b function (accession numbers: NM_001092825 and NM_001088044), while LPGDS-MO2 interfered only with LPGDS-a. A standard morpholino (Cont-MO; 5′-CCTCTTACCTCAGTTACAATTTATA-3′) was used as control. Embryos, injections and explant culture X. laevis embryos were staged according to Nieuwkoop and Faber [57] and raised in 0.1 × NAM (normal amphibian medium) [58] . This study was performed in accordance with the recommendations of the Guide for the Care and Use of Laboratory Animals of the National Institutes of Health. The procedures were approved by the Institutional Animal Care and Use Committee of New York University under animal protocol #120311. Embryos were injected in one blastomere at the two-cell stage and analysed by in situ hybridization at stage 15. Morpholino antisense oligonucleotides (40–50 ng) were injected together with 0.5 ng of β -galactosidase mRNA as a lineage tracer. Rescue experiments were performed by sequential injection of LPGDS-MO and 0.5 ng of WT or C65A mouse LPGDS mRNA. For all-trans RA and TTNPB (Sigma-Aldrich, St. Louis, MO) treatments, control and LPGDS-MO-injected embryos were incubated at stage 11 in the retinoids (0.01, 0.1, 1 and 10 μM diluted in 0.1 × NAM) and collected at stage 15 for in situ hybridization. Control and LPGDS-MO-injected embryos treated with dimethylsulphoxide were used as control. For animal explant experiments, one blastomere at the two-cell stage was injected in the animal pole region with GR or Zic1GR mRNA (0.5–1 ng), explants were dissected at the late blastula stage and immediately cultured for several hours in NAM 0.5 × plus 10 μM of dexamethasone (Sigma-Aldrich). Co-injection of 1 ng of GFP mRNA was used as a lineage tracer to identify the progeny of the injected blastomere. Dissected animal explants injected with Zic1GR mRNA were treated with 100 μM disulfiram (tetraethylthiuram disulfide) or citral (Sigma-Aldrich), two general inhibitors of alcohol and aldehyde dehydrogenases, or with 10 μM of AGN193109 (Santa Cruz Biotechnology, Dallas, TX), an RAR antagonist. In situ hybridization Embryos were fixed in MEMFA (0.1 M 3-(N-Morpholino)-propanesulfonic acid, pH 7.4, 2 mM EGTA, 1 mM MgSO 4 and 3.7% formaldehyde) and prior to in situ hybridization the β-galactosidase activity was revealed using Red-Gal (Research Organics, Cleveland, OH). Whole-mount in situ hybridization [59] was performed in 4-ml glass vials using digoxygenin (DIG)- and fluorescein isothiocyanate (FITC)-labelled antisense RNA probes (Genius Kit; Roche, Indianapolis, IN) synthesized from template complementary DNA (cDNA) encoding Zic1 (ref. 20 ), Foxi1c [18] , [19] , Six1 (ref. 17 ), Sox2 (ref. 20 ), Dmrt4 (ref. 21 ), Pax8 (ref. 22 ), Tbx2 (ref. 23 ), LPGDS (pSPORT6-LPGDS; Open Biosystems), RALDH2 (ref. 29 ) and Snail2 (ref. 16 ). Embryos were hybridized overnight at 60 o C. RNA probes were detected using an anti-DIG antibody conjugated to alkaline phosphatase (Roche) at a 1:2,000 dilution overnight at 4 o C. After several washes, the chromogenic reaction was performed overnight by incubation in BM purple (Roche). The reaction was then stopped by fixation in MEMFA and the embryos were bleached in 10% hydrogen peroxide in methanol for 48 h. For double in situ hybridization, DIG- and FITC-labelled probes were hybridized simultaneously and sequentially detected using anti-FITC- and anti-DIG alkaline phosphatase-conjugated antibodies (Roche; 1:10,000 and 1:2,000 dilution, respectively). FITC-labelled probe was visualized first using Magenta Phosphate (5-bromo-6chloro-3indoxyl phosphate; Biosynth, Itasca, IL) and after inactivation of the anti-FITC antibody by treatment with glycine (0.1 M, pH 2.2) for 30 min, the colour reaction for the DIG-labelled probe was performed using 4-toluidine salt (BCIP; Roche). The reaction was then stopped by fixation in MEMFA and the embryos were bleached in 10% hydrogen peroxide in PBS for 48 h. For in situ hybridization on sections, animal explants were fixed in 4% paraformaldehyde in PBS (Gibco, Grand Island, NY) for 1 h, embedded in Paraplast+ and 12-μm sections were collected on a glass slide and hybridized overnight at 60 o C in a humidified chamber with Foxi1c , Six1 , LPGDS or RALDH2 DIG-labelled probes. Sections were then washed in 2 × saline sodium phosphate EDTA (Invitrogen, Grand Island, NY). Probes were detected using an anti-DIG antibody conjugated to alkaline phosphatase at a 1:2,000 dilution for 2 h at room temperature. After several washes, the chromogenic reaction was performed overnight by incubation in BM purple (Roche). The reaction was stopped by fixation in MEMFA. The slides were then dehydrated and mounted in Permount (Fisher Scientific, Pittsburgh, PA) [60] . Since GFP can no longer be detected following this procedure, sections of GFP-labelled animal explants were first individually photographed and then processed for in situ hybridization. RT–PCR analysis Total RNAs were extracted from 10–15 animal explants using the RNeasy microRNA isolation kit (Qiagen, Valencia, CA). To avoid contamination from genomic DNA, the RNA samples were digested with RNase-free DNase I. RT–PCR experiments were performed using the One Step RT-PCR kit (Qiagen) according to the manufacturer’s instructions using the following primer sets: Six1 (F: 5′-CTGGAGAGCCACCAGTTCTC-3′; R: 5′-AGTGGTCTCCCCCTCAGTTT-3′; 30 cycles), Eya1 (F: 5′-ATGACACCAAATGGCACAGA-3′; R: 5′-GGGAAAACTGGTGTGCTTGT-3′; 30 cycles) and Odc (F: 5′-ACATGGCATTCTCCCTGAAG-3′; R: 5′-TGGTCCCAAGGCTAAAGTTG-3′; 25 cycles). Microarray analysis RNAs were extracted from animal explants expressing GR, Pax3GR, Zic1GR or a combination of Pax3GR and Zic1GR using the RNeasy microRNA isolation kit. During the extraction procedure, the samples were treated with DNase I to eliminate possible genomic DNA contamination. The amount of isolated RNA was quantified using a spectrophotometer. Extracted RNAs (five replicate for each injection set) were used for the microarray experiment. Probe labelling, hybridization and initial data analysis were performed at the University of Pennsylvania Microarray Facility. Around 0.1–0.2 μg total RNA was converted into first-strand cDNA using Superscript II reverse transcriptase primed by a poly(T) oligomer that incorporates the T7 promoter. Second-strand cDNA synthesis is followed by in vitro transcription for linear amplification of each transcript and incorporation of biotinylated nucleotides. The cRNA products were fragmented to 200 nucleotides or less, heated at 99 °C for 5 min and hybridized for 16 h at 45 °C to a GeneChip Xenopus laevis Genome 2.0 Array (Affymetrix, Cleveland, OH). Hybridized arrays were processed by the GeneChip Fluidics system, and scanned in the GeneChip Scanner. Probe intensities were exported in cel files using GCOS software (Affymetrix). Subsequent quantification of expression levels and statistical identification of differentially regulated genes was performed using Partek Genomics Suite (Partek, Inc., St. Louis, MO). Normalized, log2-transformed probeset intensities were calculated using GeneChip Robust Multiarray Averaging (GC-RMA). Analysis of variance with multiple testing corrections was used to determine P values for likelihood of differential expression, based on reproducibility in five replicates to identify cDNAs both activated by Zic1GR and repressed in Zic1GR/Pax3GR samples. Pairwise comparisons yielding fold changes were performed between these conditions. The microarray data have been deposited in the GEO database under the accession number GSE68546. PGD2 signalling inhibitors and treatment To interfere with PGD2 signalling pathway, we used well-characterized pharmacological inhibitors: AT-56 (Tocris Bioscience, Minneapolis, MN) to block LPGDS enzymatic activity, and two antagonists of PGD2 receptors, BWA868C (Cayman Chemical, Ann Arbor, MI) specific for DP1 and ramatroban (Sigma-Aldrich) specific for DP2. For treatment, embryos at stage 11 devoid of the vitelline membrane were incubated in the presence of the inhibitors (1, 10 and 100 μM in NAM 0.1 × ), collected at stage 15 and processed for in situ hybridization. Dimethylsulphoxide-treated embryos were used as control. Imaging Images were captured using an Olympus SZX9 microscope and a QImaging Micro Publisher 3.3 RTV camera. Images from sections of animal explants were obtained on a Nikon SMZ1500 microscope equipped with a Nikon Ds-U3 camera. Composite images were assembled using Adobe Photoshop. In some experiments RFP mRNA was injected as a lineage tracer, in place of GFP mRNA and for consistency, the images were then digitally coloured (green) using ImageJ; this applies specifically to Fig. 5c (RALDH2; lower panels). Accession codes: The microarray data have been deposited in the GEO database under the accession number GSE68546 . How to cite this article: Jaurena, M. B. et al. Zic1 controls placode progenitor formation non-cell autonomously by regulating retinoic acid production and transport. Nat. Commun. 6:7476 doi: 10.1038/ncomms8476 (2015).